Tousled-like kinases phosphorylate Asf1 to promote histone supply during DNA replication During DNA replication, nucleosomes are rapidly assembled on newly synthesized DNA to restore chromatin organization. Asf1, a key histone H3-H4 chaperone required for this process, is phosphorylated by Tousled-like kinases (TLKs). Here, we identify TLK phosphorylation sites by mass spectrometry and dissect how phosphorylation has an impact on human Asf1 function. The divergent C-terminal tail of Asf1a is phosphorylated at several sites, and this is required for timely progression through S phase. Consistent with this, biochemical analysis of wild-type and phospho-mimetic Asf1a shows that phosphorylation enhances binding to histones and the downstream chaperones CAF-1 and HIRA. Moreover, we find that TLK phosphorylation of Asf1a is induced in cells experiencing deficiency of new histones and that TLK interaction with Asf1a involves its histone-binding pocket. We thus propose that TLK signalling promotes histone supply in S phase by targeting histone-free Asf1 and stimulating its ability to shuttle histones to sites of chromatin assembly. In S phase of the cell cycle, DNA must be accurately duplicated and its organization into chromatin reproduced to maintain genetic and epigenetic information. During DNA replication, chromatin organization is disrupted ahead of the replisome and restored behind, on the two daughter strands [1] , [2] , [3] . To maintain nucleosomal density, parental histone recycling must be complemented by deposition of newly synthesized histones. Duplication of chromatin thus necessitates an efficient supply of new histones, which is partly achieved by the coordination of canonical histone biosynthesis with DNA replication [4] . Before their incorporation into chromatin, soluble histones are handled by histone chaperones. Asf1 is a key histone H3-H4 chaperone [5] and loss of Asf1 function causes severe replication defects and loss of chromatin integrity [6] , [7] , [8] , [9] . Asf1 participates in replication-coupled nucleosome assembly by shuttling newly synthesized histone H3.1-H4 dimers to sites of ongoing replication. This process most likely relies on histone transfer between different chaperone complexes dedicated to histone acetylation (RbAp46-HAT1), histone nuclear import (Asf1, Importin-4) and histone storage (NASP) [6] , [10] , [11] , [12] , [13] . In the nucleus, Asf1 donates histones H3.1-H4 to CAF-1 (refs 5 , 14 , 15 , 16 ), which through interaction with PCNA deposits histones onto newly synthesized DNA [17] , [18] . Furthermore, Asf1 may contribute to parental histone recycling through its association with the replicative helicase MCM2-7 (refs 11 , 19 ). If replication is arrested in response to genotoxic insults, Asf1 acts as a buffer to store excess histones that cannot be incorporated into chromatin [6] , [11] . In addition to its replication-coupled functions, Asf1 supplies replacement histone H3.3-H4 dimers to HIRA for replication-independent chromatin assembly [20] , [21] . The mechanisms that control Asf1 activity and direct it towards distinct assembly pathways are not well understood. In humans, there are two Asf1 isoforms, Asf1a and Asf1b, with largely redundant roles in S phase [6] , [19] , [22] . Both isoforms can deliver histones to CAF-1 for DNA synthesis-coupled chromatin assembly in vitro [6] , [15] , and only co-depletion of Asf1a and Asf1b arrests cells in S phase [6] , [19] . Both isoforms bind histone H3.1-H4 and H3.3-H4 in vivo [20] , but Asf1a appears to be the main histone donor for HIRA [20] , [21] , [23] . Consistent with this, Asf1b is expressed only in proliferating cells [22] , [24] , while Asf1a is expressed also in quiescence [22] . The N-terminal domain, highly conserved between Asf1a and Asf1b, forms a β-barrel structure [25] , [26] with a hydrophobic groove accommodating the H3-H4 dimer and a B-domain-binding pocket placed on the opposite side [25] , [27] , [28] . The latter serves as a docking site for the downstream chaperones HIRA and CAF-1 (refs 21 , 26 ). How histone transfer occurs is poorly understood, but it may involve conformational changes in both the H3-H4 dimer and within Asf1 itself [29] , [30] . The C-terminal tail of Asf1 is unstructured and highly divergent among species and the Asf1a and Asf1b isoforms. The tail of yeast Asf1 contains long stretches of acidic amino acids that contribute to histone binding [9] , [26] , [31] . In higher eukaryotes, Asf1 homologues are subject to regulation by serine/threonine kinases of the Tousled-like family (TLKs) [32] , but the functional implications of phosphorylation have so far remained elusive. However, as the C-terminal acidic stretches are largely lost in metazoan Asf1 homologues, it has been speculated that TLK phosphorylation somehow would compensate for this [33] . TLKs are S phase active kinases [34] , which are rapidly inactivated in response to genotoxic stress through phosphorylation by the checkpoint kinase Chk1 (refs 35 , 36 ). In Drosophila and C. elegans , TLK deletion causes developmental arrest due to serious defects in chromatin organization and replication [37] , [38] , while TLK depletion in human cells leads to chromosome segregation defects and aneuploidy [39] . Genetic analysis in flies argues that the deregulation of Asf1 function is at least partly responsible for these defects [37] , although the underlying mechanism remains unclear. Here, we dissect how TLK phosphorylation regulates Asf1 function. Using mass spectrometry, we identify multiple TLK phosphorylation sites in the C-terminal tails of human Asf1a and Asf1b. Analyses of phosphorylation-deficient and phospho-mimetic mutants reveal that TLK phosphorylation of Asf1 promotes S phase progression and facilitates its interaction with histones and downstream chaperones in vivo . Consistent with these findings, Asf1 phosphorylation peaks in S phase and is further enhanced when the demand for new histones is high due to inhibition of histone biosynthesis. Taken together, our results suggest that TLK phosphorylates histone-free Asf1 to promote provision of histones for chromatin assembly. Identification of TLK1 phosphorylation sites in Asf1 Mass spectrometry (LC-MS/MS) was used to map phosphorylation sites in Asf1a and Asf1b phosphorylated in vitro by TLK1 and in vivo in HeLa cells. We phosphorylated recombinant Asf1a and Asf1b in vitro with recombinant myc-TLK1 and isolated potential phosphorylated forms of Asf1 based on their slower migration in SDS-PAGE ( Supplementary Figs 1a and 2a ). Because of the low number of trypsin cleavage sites and high frequency of serines and threonines in the C-terminal tail of Asf1, the low specificity protease thermolysin was primarily used for digestion and precise mapping of the individual phosphorylation sites (for details see Methods). Out of twelve serine/threonines in the Asf1a C-terminal tail, we identified a total of four phosphorylation sites (S166, S175, S192 and S199) ( Fig. 1a and Supplementary Fig. 1 ). In the tail of Asf1b, we found two phosphorylation sites (S169 and S198) ( Fig. 1a and Supplementary Fig. 2 ). 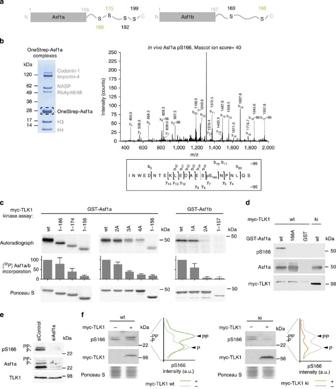Figure 1: Identification of TLK1 phosphorylation sites in Asf1a and Asf1b. (a) TLK1 phosphorylation sites in Asf1a and Asf1b mapped by mass spectrometry. Sites identifiedin vitroare in black, sites detected bothin vitroandin vivoare green. For details see Methods andSupplementary Figs 1–3. N-terminal domains are depicted as rectangles, and C-terminal tails as lines. (b) (Left) OneStrep-Asf1a complexes isolated from asynchronous HeLa S3 cells for LC-MS/MS of Asf1a (boxed). (Right) MS/MS spectra of the Asf1a pS166 peptide. Observed b- and y-ions, and those resulting from the neutral loss of H3PO4(−98 Da) are indicated. (c)In vitrophosphorylation of GST-Asf1 by recombinant myc-TLK1. Asf1a: wt (wild-type, amino acid 1–204), 1–186 and 1–174 (tail truncations), 1–156 (tail deletion), 2A (S166A, S175A), 3A (S166A, S175A, S192A), 4A (S166A, S175A, S192A, S199A). Asf1b: wt (amino acid 1–202), 1–157 (tail deletion), 1A (S198A), 2A (S169A, S198A). [32P] incorporation was quantified on a phosphoimager in 3–5 independent experiments; error bars represent s.d. (d) Test of Asf1a pS166 antibodies against GST-Asf1a wt or S166A pre-incubated with myc-TLK1 wild-type (wt) or kinase-inactive (ki) in kinase reactions. (e) Western blot of pS166 in siRNA treated U-2-OS cells. (f) Analysis of Asf1a pS166 in cells expressing myc-TLK1 wt or ki. Graphs show pS166 signals as a function of distance. P and PP denote different phosphorylation states. One representative experiment out of two biological replicas is shown. Figure 1: Identification of TLK1 phosphorylation sites in Asf1a and Asf1b. ( a ) TLK1 phosphorylation sites in Asf1a and Asf1b mapped by mass spectrometry. Sites identified in vitro are in black, sites detected both in vitro and in vivo are green. For details see Methods and Supplementary Figs 1–3 . N-terminal domains are depicted as rectangles, and C-terminal tails as lines. ( b ) (Left) OneStrep-Asf1a complexes isolated from asynchronous HeLa S3 cells for LC-MS/MS of Asf1a (boxed). (Right) MS/MS spectra of the Asf1a pS166 peptide. Observed b- and y-ions, and those resulting from the neutral loss of H 3 PO 4 (−98 Da) are indicated. ( c ) In vitro phosphorylation of GST-Asf1 by recombinant myc-TLK1. Asf1a: wt (wild-type, amino acid 1–204), 1–186 and 1–174 (tail truncations), 1–156 (tail deletion), 2A (S166A, S175A), 3A (S166A, S175A, S192A), 4A (S166A, S175A, S192A, S199A). Asf1b: wt (amino acid 1–202), 1–157 (tail deletion), 1A (S198A), 2A (S169A, S198A). [ 32 P] incorporation was quantified on a phosphoimager in 3–5 independent experiments; error bars represent s.d. ( d ) Test of Asf1a pS166 antibodies against GST-Asf1a wt or S166A pre-incubated with myc-TLK1 wild-type (wt) or kinase-inactive (ki) in kinase reactions. ( e ) Western blot of pS166 in siRNA treated U-2-OS cells. ( f ) Analysis of Asf1a pS166 in cells expressing myc-TLK1 wt or ki. Graphs show pS166 signals as a function of distance. P and PP denote different phosphorylation states. One representative experiment out of two biological replicas is shown. Full size image Next, we addressed whether Asf1 (a and b) phosphorylation could be detected in vivo at the sites identified in vitro . We took advantage of HeLa S3 cells stably expressing OneStrep-tagged Asf1a and Asf1b [19] to purify proteins for mass spectrometry. For Asf1a, phosphorylations occurring at S166 and S175 were identified ( Fig. 1b and Supplementary Fig. 3a ). For Asf1b, we used cells synchronized in S phase and identified phosphorylations on S198 and T179 ( Supplementary Fig. 3b ). Given that pT179 was not identified after extensive phosphorylation of Asf1b with myc-TLK1 in vitro , we believe that this residue is probably targeted by other kinases in vivo . To further validate the identified phosphorylation sites, we tested Asf1a and Asf1b truncation and serine to alanine (S/A) mutants in a myc-TLK1 kinase assay. The level of phosphorylation decreased gradually upon shortening of the C-terminal tail of Asf1a, and removal of the entire tail reduced phosphorylation by 85% compared with the wild type ( Fig. 1c , compare 1–156 and wt). Single serine to alanine substitutions as well as simultaneous mutation of the sites identified in vivo (Asf1a pS166, pS175) had a moderate effect ( Fig. 1c , see Asf1a 2A; Supplementary Fig. 4a ). However, mutation of all four sites identified in vitro reduced phosphorylation to the same extent as removing the full Asf1a tail ( Fig. 1c , compare Asf1a 4A and 1–156). Similarly, substituting both serines identified in vitro (Asf1b pS169, pS198) or truncation of the C-terminal tail (Asf1b 1–157) eliminated phosphorylation of Asf1b ( Fig. 1c , compare Asf1b 2A, 1–157 and wt). Taken together, our mapping analysis argues that TLKs can target four sites in Asf1a and two sites in Asf1b, all located within the divergent C-terminal tails. To study Asf1a phosphorylation in vivo , we generated antibodies against all sites in Asf1a and Asf1b that had reasonable immunogenic properties (Asf1a pS166, pS175, pS192; Asf1b pS169). Of these, only the antibody against Asf1a pS166 showed high specificity. It recognized wild-type Asf1a phosphorylated by myc-TLK1 in vitro but not the S166A mutant or the unphosphorylated wild-type protein ( Fig. 1d ). In total cell lysates, the pS166 antibody detected two bands, which correspond to slow migrating forms of Asf1a ( Fig. 1e ). It should be noted that the resolution of these phospho-forms depends on the SDS-PAGE conditions and are not always easily discernible. Importantly, the pS166 signal was enhanced upon overexpression of wild-type myc-TLK1, while kinase-inactive (ki) myc-TLK1 markedly reduced both phospho-forms ( Fig. 1f ). Thus, the pS166 antibody specifically detects TLK phosphorylation of Asf1a at S166, and the two bands probably represent differentially phosphorylated forms of Asf1a that have pS166 in common. Asf1a pS166 is nuclear and peaks during DNA synthesis TLKs are hyperactive in S phase [34] and rapidly inactivated upon DNA damage or replication stress through direct phosphorylation by Chk1 (refs 35 , 36 ). We thus used the pS166 antibody to monitor TLK1 phosphorylation of Asf1a during the cell cycle and after treatment with replication inhibitors. Analysis of synchronized U-2-OS cells showed that Asf1a S166 phosphorylation peaks in mid S phase and decreases in late S and G2 phase ( Fig. 2a ). Consistent with this, immunofluorescence analysis revealed nuclear Asf1a pS166 staining in most replicating cells marked by EdU ( Fig. 2b ). However, a fraction of pS166-positive cells did not incorporate EdU. While some of these might represent cells at the G1/S transition, others were in mitosis when TLK2 is known to have moderate activity [32] , [34] . No staining was seen in Asf1a-depleted cells, verifying the specificity of the antibody ( Fig. 2b ). This confirms that the slow migrating phospho-forms of Asf1a previously observed in S phase [32] reflect TLK-mediated phosphorylation. Inhibition of DNA replication by hydroxyurea (HU) reduced Asf1 S166 phosphorylation by 60–85% within 1 h, as shown by western blot, immunoprecipitation and immunostaining ( Fig. 2a,c and d ). Concomitant treatment with the Chk1 inhibitor UCN-01 partially rescued Asf1 pS166 ( Fig. 2c ). Yet, the effect of checkpoint abrogation was modest, suggesting that checkpoint-independent events may contribute to the loss of Asf1 phosphorylation upon a replication block (see discussion). Nonetheless, Chk1 inhibition augmented Asf1a pS166 in unperturbed S phase cells ( Fig. 2c,d ), indicating that Asf1 phosphorylation, similar to TLK activity [35] , is controlled by basal Chk1 activity in S phase. 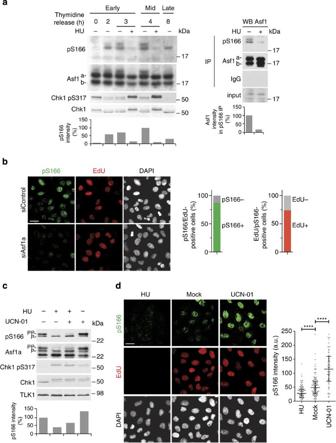Figure 2: Asf1a pS166 is nuclear and peaks during ongoing DNA synthesis. (a) U-2-OS cells were synchronized by a thymidine block at the G1/S boundary and released into S-phase (early S, mid S, late S/G2). Parallel cultures were treated for one hour with HU, as indicated. (Left) pS166 western blot. (Right) Immunoprecipitation with pS166 and Asf1 (a and b) antibodies followed by western blot for Asf1. Graphs show relative pS166 or Asf1 signal intensities. One representative experiment out of two biological replicas is shown. (b) Immunofluorescence analysis of Asf1a pS166 in siRNA treated U-2-OS cells. Replicating cells were labelled with EdU. Graphs depict the percentage of pS166-positive/negative cells in the EdU-positive population and vice versa. More than 120 cells per sample were analysed. Scale bar, 32 μm. (c) U-2-OS cells synchronized in early S phase as in (a) were treated with HU and/or UCN-01 for 1 h. Relative pS166 signal intensities are depicted in the graph. One representative experiment out of two biological replicas is shown. (d) Immunofluorescence analysis of Asf1a pS166 in cells treated as in (c). Replicating cells were labelled with EdU. Scale bar, 32 μm. Graph shows pS166 intensities, where median and interquartile range are indicated,n>70, ****P<0.0001 (unpairedt-test). P and PP denote different Asf1a phosphorylation states. Figure 2: Asf1a pS166 is nuclear and peaks during ongoing DNA synthesis. ( a ) U-2-OS cells were synchronized by a thymidine block at the G1/S boundary and released into S-phase (early S, mid S, late S/G2). Parallel cultures were treated for one hour with HU, as indicated. (Left) pS166 western blot. (Right) Immunoprecipitation with pS166 and Asf1 (a and b) antibodies followed by western blot for Asf1. Graphs show relative pS166 or Asf1 signal intensities. One representative experiment out of two biological replicas is shown. ( b ) Immunofluorescence analysis of Asf1a pS166 in siRNA treated U-2-OS cells. Replicating cells were labelled with EdU. Graphs depict the percentage of pS166-positive/negative cells in the EdU-positive population and vice versa. More than 120 cells per sample were analysed. Scale bar, 32 μm. ( c ) U-2-OS cells synchronized in early S phase as in ( a ) were treated with HU and/or UCN-01 for 1 h. Relative pS166 signal intensities are depicted in the graph. One representative experiment out of two biological replicas is shown. ( d ) Immunofluorescence analysis of Asf1a pS166 in cells treated as in ( c ). Replicating cells were labelled with EdU. Scale bar, 32 μm. Graph shows pS166 intensities, where median and interquartile range are indicated, n >70, **** P <0.0001 (unpaired t -test). P and PP denote different Asf1a phosphorylation states. Full size image TLK1 phosphorylation of Asf1a facilitates S-phase progression To explore the role of Asf1 phosphorylation in S phase, we established U-2-OS Flp-In cells conditionally expressing FLAG-HA-Asf1a (e-Asf1a) wild-type (wt), a phosphorylation deficient (4A) mutant or a phospho-mimetic mutant (4D), all rendered insensitive to siRNAs targeting endogenous Asf1a. We chose to mutate all four sites identified with high confidence in vitro , since this reduced TLK phosphorylation by 85% similar to removing the whole C-terminal tail ( Fig. 1c ). A recent study found that TLK2 can phosphorylate Asf1a at S192 in vitro and proposed that phosphorylation of this single site stabilizes Asf1a by preventing proteasomal degradation [40] . We therefore tested the stability of our Asf1a phospho-mimetic (4D) and phosphorylation deficient (4A) mutants in cycloheximide (CHX)-treated cells. We did not observe significant differences in stability ( Supplementary Fig. 4b ). However, we noted that CHX treatment strongly stimulated Asf1 phosphorylation ( Supplementary Figs 4b , 6b ), which due to the mobility shift might influence stability measurements of the wild-type protein. Figure 6: TLK1 localizes to replication sites and phosphorylates histone-free Asf1. ( a ) In vitro binding assay. Recombinant Asf1a wild-type (wt) or histone-binding mutant (V94R) was incubated with myc-TLK1 wild-type (wt) or kinase-inactive (ki) isolated from insect cells. 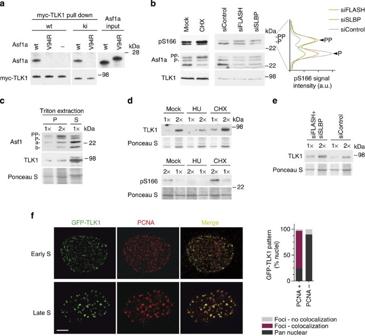Figure 6: TLK1 localizes to replication sites and phosphorylates histone-free Asf1. (a)In vitrobinding assay. Recombinant Asf1a wild-type (wt) or histone-binding mutant (V94R) was incubated with myc-TLK1 wild-type (wt) or kinase-inactive (ki) isolated from insect cells. (b) Western blot of Asf1a phosphorylation in S phase cells treated with CHX for one hour or siRNAs against FLASH and SLBP (siFLASH, siSLBP). Graph was generated as inFig. 1f. One representative experiment out of two biological replicas is shown. (c) Distribution of TLK1 and Asf1 between the Triton soluble (S) fraction and chromatin pellet (P) in S phase cells. P and PP denote different Asf1a phosphorylation states. (d,e) Analysis of TLK1 and Asf1a pS166 in the chromatin pellet in cells treated with HU and CHX for one hour (d) or siRNAs against FLASH and SLBP (siFLASH+siSLBP) (e). (f) GFP-TLK1 localization analysed in conditional U-2-OS cells by co-staining with PCNA after pre-extraction of soluble proteins with Triton. Representative images of early and late S phase cells are shown. Scale bar, 5 μm. The graph shows quantification of GFP-TLK1 localization patterns in PCNA-positive (+) and PCNA-negative (−) cells. One representative experiment out of two biological replicas is shown (n>100). ( b ) Western blot of Asf1a phosphorylation in S phase cells treated with CHX for one hour or siRNAs against FLASH and SLBP (siFLASH, siSLBP). Graph was generated as in Fig. 1f . One representative experiment out of two biological replicas is shown. ( c ) Distribution of TLK1 and Asf1 between the Triton soluble (S) fraction and chromatin pellet (P) in S phase cells. P and PP denote different Asf1a phosphorylation states. ( d , e ) Analysis of TLK1 and Asf1a pS166 in the chromatin pellet in cells treated with HU and CHX for one hour ( d ) or siRNAs against FLASH and SLBP (siFLASH+siSLBP) ( e ). ( f ) GFP-TLK1 localization analysed in conditional U-2-OS cells by co-staining with PCNA after pre-extraction of soluble proteins with Triton. Representative images of early and late S phase cells are shown. Scale bar, 5 μm. The graph shows quantification of GFP-TLK1 localization patterns in PCNA-positive (+) and PCNA-negative (−) cells. One representative experiment out of two biological replicas is shown ( n >100). Full size image Overexpression of either Asf1a wild-type or the phospho-mutants did not significantly perturb the cell cycle ( Supplementary Fig. 4c ). We thus asked whether the mutants could substitute for endogenous Asf1a and rescue cells arrested in S phase due to co-depletion of Asf1a and Asf1b ( Fig. 3 ). We chose to deplete both isoforms, as single depletions do not efficiently block S phase progression [22] . Western blotting confirmed the efficient depletion of endogenous Asf1 (a and b) and equal expression of e-Asf1a proteins ( Fig. 3a ). In the absence of Asf1 (a and b), approximately 50% of the cells were in S phase, as compared with 25% of the control cells ( Fig. 3b,c ). Short-term expression of wild-type e-Asf1a reduced the number of the S phase cells to 35%, and the phospho-mimetic mutant (4D) had similar or better rescue efficiency ( Fig. 3b ). In contrast, the e-Asf1a 4A mutant showed significantly lower rescue activity ( Fig. 3b,c , Supplementary Fig. 4d ). Similarly, complementation of synchronized cells illustrated that phospho-mimetic Asf1a accelerated S-phase progression most efficiently, while the phospho-deficient mutant was inferior to wild-type Asf1a ( Fig. 3d,e , Supplementary Fig. 4e,f ). 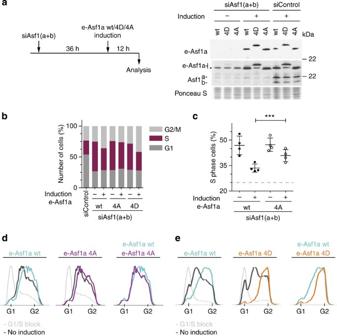This indicates that TLK phosphorylation promotes Asf1 function in S phase. Figure 3: TLK1 phosphorylation of Asf1a facilitates S phase progression. (a) (Left) Experimental design for complementation analysis. (Right) Western blot showing induction of siRNA-resistant forms of e-Asf1a wt/4D/4A after depletion of endogenous Asf1 a and b (siAsf1(a+b)). *, unspecific band. (b) Quantification of cell cycle distribution. Cell cycle profiles are shown inSupplementary Fig. 4b. (c) Quantification of S phase cells in 4 independent experiments comparing the complementation efficiency for e-Asf1a wt vs. 4A. The mean with s.d is shown; ***P=0.0008 (unpaired t test). The dashed line shows average percentage of S phase cells in siControl cells. (d,e) Complementation analysis in synchronized cells. Complementation of endogenous Asf1 (a and b) was assessed 9 h after release from a G1/S arrest. Asf1a proteins were expressed at similar levels and endogenous Asf1 (a and b) were efficiently depleted (Supplementary Fig. 4e,f).Light grey lines, control cells in G1/S;dark grey lines,Asf1 (a and b)-depleted cells without induction;colored lines, Asf1 (a and b) depleted cells complemented with e-Asf1a wt (blue), 4A (purple) and 4D (orange). Figure 3: TLK1 phosphorylation of Asf1a facilitates S phase progression. ( a ) (Left) Experimental design for complementation analysis. (Right) Western blot showing induction of siRNA-resistant forms of e-Asf1a wt/4D/4A after depletion of endogenous Asf1 a and b (siAsf1(a+b)). *, unspecific band. ( b ) Quantification of cell cycle distribution. Cell cycle profiles are shown in Supplementary Fig. 4b . ( c ) Quantification of S phase cells in 4 independent experiments comparing the complementation efficiency for e-Asf1a wt vs. 4A. The mean with s.d is shown; *** P =0.0008 (unpaired t test). The dashed line shows average percentage of S phase cells in siControl cells. ( d , e ) Complementation analysis in synchronized cells. Complementation of endogenous Asf1 (a and b) was assessed 9 h after release from a G1/S arrest. Asf1a proteins were expressed at similar levels and endogenous Asf1 (a and b) were efficiently depleted ( Supplementary Fig. 4e,f ). Light grey lines , control cells in G1/S; dark grey lines, Asf1 (a and b)-depleted cells without induction; colored lines , Asf1 (a and b) depleted cells complemented with e-Asf1a wt (blue), 4A (purple) and 4D (orange). Full size image Phosphorylation promotes complex formation with histones Next we explored whether phosphorylation influences the properties of Asf1 as a histone chaperone by comparing complex composition of wild-type Asf1a against the phosphorylation-deficient (4A) and phospho-mimetic (4D) mutants. We used our conditional cell lines to purify complexes from cells synchronized in mid S phase. Comparison of cytosolic complexes, representing highly soluble cytoplasmic and nuclear Asf1 (ref. 11 ), showed that the phospho-mimetic Asf1a mutant binds more histone H3, new histone H4 acetylated at lysine 12, Importin-4, NASP and RbAp46/48 than wild-type Asf1a ( Fig. 4a ). Importin-4, NASP and RbAp46/48 form a complex with Asf1 through mutual binding to histone H3-H4 (ref. 11 ), and their abundances are thus expected to mirror histone binding as we observe. Previous work has shown that Asf1 distributes into a histone-bound multi-chaperone complex and a histone-free form in cytosolic extracts from S phase cells [6] . Analysis of the phospho-mutants by gel-filtration demonstrated a clear shift of the Asf1a phospho-mimetic mutant (4D) towards the histone-bound complex relative to the wild-type and 4A proteins ( Fig. 4b , Supplementary Fig. 5a ). Consistent with this, S166 phosphorylation on endogenous Asf1a could also be detected in the histone-bound complex ( Supplementary Fig. 5b ). Moreover, TLK1 phosphorylation of GST-Asf1a enhanced histone H3-H4 binding in cell extracts ( Supplementary Fig. 5c ). These data imply that phosphorylated Asf1 might bind soluble cellular histones more efficiently. Kinetic rate constants between recombinant Asf1a and immobilized histone H3-H4 in vitro were therefore determined by surface plasmon resonance ( Supplementary Fig. 6 ). The derived rate constants translates into a very high affinity ( K d =46±24 pM, Supplementary Fig. 6 ) for the interaction between wild-type Asf1a and histones, which align very well with previous data recorded at equilibrium [30] . However, using these experimental conditions we could not detect significant differences between wild-type Asf1a and the phospho-mimetic mutant. It is, nevertheless, possible that the electrostatic immobilization of H3-H4 on the sensor chip sterically prevents an interaction with the acid tail of phospo-mimetic Asf1, thus providing a suboptimal surrogate for cellular histones. We therefore devised a competition assay to compare the binding of recombinant wild-type and phospho-mimetic proteins to histones in a cell extract. Recombinant Asf1a wild-type and phospho-mimetic mutant (4E) were added together to an extract of HeLa S3 cells expressing H3.1-HA-FLAG (e-H3.1). Upon isolation of e-H3.1 complexes, we found a significant enrichment of the phospho-mimetic mutant relative to recombinant wild-type Asf1a ( Fig. 4c ). Importantly, this was paralleled by a larger depletion of the phospho-mimetic mutant from the unbound fraction. 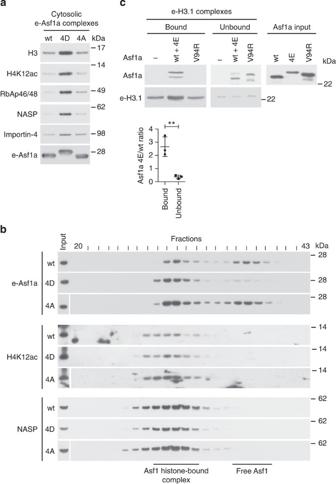Asf1a containing a mutated histone-binding pocket (V94R) [25] did not bind histones in the extract. Figure 4: Phosphorylation enhances Asf1 binding to soluble cellular histones. (a) Western blot analysis of e-Asf1a complexes isolated from conditional cell lines expressing e-Asf1a wt/4D/4A. Cytosolic complexes were obtained from cells released into mid-S phase from a thymidine block. (b) Gel-filtration analysis of cytosolic extracts from S phase cells conditionally expressing e-Asf1a wt/4D/4A. Similar induction of e-Asf1a wt/4D/4A was verified (Supplementary Fig. 5a). Two distinct Asf1 complexes are indicated. (c)In vitrocompetition assay. Whole-cell extracts of HeLa S3 cells expressing H3.1-HA-FLAG20were pre-incubated with mixture of recombinant Asf1a wt and phospho-mimetic (4E) mutant or with Asf1a V94R. e-H3.1 complexes were purified and binding of recombinant Asf1a assessed taking advantage of the difference in mobility between wt and 4E. The ratio of Asf1a 4E relative to wt in the bound and unbound fractions was quantified in three independent experiments as depicted in the graph. The mean with s.d is shown, **P=0.0063 (unpairedt-test). Figure 4: Phosphorylation enhances Asf1 binding to soluble cellular histones. ( a ) Western blot analysis of e-Asf1a complexes isolated from conditional cell lines expressing e-Asf1a wt/4D/4A. Cytosolic complexes were obtained from cells released into mid-S phase from a thymidine block. ( b ) Gel-filtration analysis of cytosolic extracts from S phase cells conditionally expressing e-Asf1a wt/4D/4A. Similar induction of e-Asf1a wt/4D/4A was verified ( Supplementary Fig. 5a ). Two distinct Asf1 complexes are indicated. ( c ) In vitro competition assay. Whole-cell extracts of HeLa S3 cells expressing H3.1-HA-FLAG [20] were pre-incubated with mixture of recombinant Asf1a wt and phospho-mimetic (4E) mutant or with Asf1a V94R. e-H3.1 complexes were purified and binding of recombinant Asf1a assessed taking advantage of the difference in mobility between wt and 4E. The ratio of Asf1a 4E relative to wt in the bound and unbound fractions was quantified in three independent experiments as depicted in the graph. The mean with s.d is shown, ** P =0.0063 (unpaired t -test). Full size image To address whether phosphorylation also affected the interaction with Asf1 downstream chaperones, CAF-1 and HIRA, we analysed complexes from nuclear extracts made by high-salt extraction of chromatin [19] . The nuclear e-Asf1a 4D complexes showed increased association to both non-nucleosomal histone H3-H4 and the two downstream chaperones CAF-1 and HIRA ( Fig. 5a ). To corroborate these findings, we used SILAC-based mass spectrometry to quantitatively compare the composition of wild-type and phospho-mimetic Asf1a complexes isolated from whole-cell extracts. This approach confirmed our western blot data, showing up to twofold more histone H3-H4, Importin-4, NASP, RbAb46 and HIRA in e-Asf1a 4D complexes ( Fig. 5b ). We did not detect CAF-1 in the SILAC analysis, likely reflecting that this interaction is weak compared with HIRA binding [21] . However, analysis of Asf1b complexes showed that, although histone H3-H4 binding was not markedly changed, the phospho-mimetic mutations clearly favoured association with CAF-1 ( Fig. 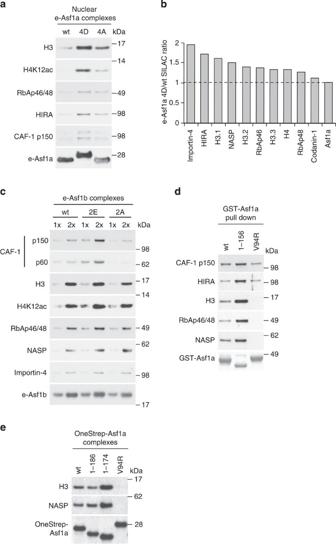5c ). Figure 5: Phosphorylation promotes Asf1 complex formation with downstream chaperones. (a) Western blot analysis of e-Asf1a complexes isolated from conditional cell lines expressing e-Asf1a wt/4D/4A. Nuclear extracts were prepared from cells synchronized as inFig. 4a. (b) SILAC-based proteomic analysis of e-Asf1a 4D and wt complexes. Complexes were isolated from whole extracts of conditional cells grown in heavy (e-Asf1a 4D) and light (e-Asf1a wt) amino acids, mixed in a 1:1 ratio and analysed by mass spectrometry. The relative enrichment in e-Asf1a 4D versus wt complexes of known binding partners is indicated with raw ratios. A dashed line indicates no enrichment. The result of a representative experiment out of three biological replicates is shown. (c) Complexes containing Flag-HA-Asf1b (e-Asf1b) wt, phospho-mimetic (2E: S169E and S198E) and phosphorylation-deficient (2A: S169A and S198A) mutants were affinity purified from whole cell extracts of transiently transfected U-2-OS cells. (d) Tail-deletion augments Asf1 binding to soluble histones. Pull-down using GST-Asf1a full length (wt), truncated (1–156) or histone-binding (V94R) mutant as bait in U-2-OS cell extracts. (e) Complexes containing OneStrep-Asf1a wt, truncations (1–174, 1–186) or V94R mutant purified from whole-cell extracts of transiently transfected U-2-OS cells. Figure 5: Phosphorylation promotes Asf1 complex formation with downstream chaperones. ( a ) Western blot analysis of e-Asf1a complexes isolated from conditional cell lines expressing e-Asf1a wt/4D/4A. Nuclear extracts were prepared from cells synchronized as in Fig. 4a . ( b ) SILAC-based proteomic analysis of e-Asf1a 4D and wt complexes. Complexes were isolated from whole extracts of conditional cells grown in heavy (e-Asf1a 4D) and light (e-Asf1a wt) amino acids, mixed in a 1:1 ratio and analysed by mass spectrometry. The relative enrichment in e-Asf1a 4D versus wt complexes of known binding partners is indicated with raw ratios. A dashed line indicates no enrichment. The result of a representative experiment out of three biological replicates is shown. ( c ) Complexes containing Flag-HA-Asf1b (e-Asf1b) wt, phospho-mimetic (2E: S169E and S198E) and phosphorylation-deficient (2A: S169A and S198A) mutants were affinity purified from whole cell extracts of transiently transfected U-2-OS cells. ( d ) Tail-deletion augments Asf1 binding to soluble histones. Pull-down using GST-Asf1a full length (wt), truncated (1–156) or histone-binding (V94R) mutant as bait in U-2-OS cell extracts. ( e ) Complexes containing OneStrep-Asf1a wt, truncations (1–174, 1–186) or V94R mutant purified from whole-cell extracts of transiently transfected U-2-OS cells. Full size image The unstructured C-terminal tails of Asf1a and Asf1b are approximately 50 amino acids long and extrude from the globular domain between the histone-binding pocket and the B-domain binding surface [25] , [26] , [27] , [28] . To address how the tail might influence interactions at these sites, we performed a series of pull-down experiments using truncated versions of GST-Asf1a. Tail-less Asf1a retrieved histones, histone-dependent interactors (NASP, RbAp46/48) as well as CAF-1 and HIRA more efficiently than the full-length protein from HeLa S3 cell extracts ( Fig. 5d ). Furthermore, isolation of complexes from transiently transfected cells revealed that removal of only 30 amino acids from the Asf1a tail was sufficient to improve complex formation with histones and NASP ( Fig. 5e ). Histone deficiency induces TLK phosphorylation of Asf1 In our GST pull-down experiments, we noted that tailless Asf1a bound efficiently to TLK1 ( Supplementary Fig. 7a ). Furthermore, we found that an intact histone-binding pocket, but not the B-domain binding site, is required to pull-down TLK1 from cell extracts ( Supplementary Fig. 7a ). This suggests that TLK1 either interacts directly with the histone-binding pocket in Asf1 or binds via histone H3-H4. Consistent with the first scenario, in vitro binding reactions with recombinant proteins showed that myc-TLK1 failed to bind Asf1a V94R ( Fig. 6a ). This implies that TLK1 docks onto Asf1 via the histone-binding pocket and thus predicts that histone-free Asf1 would be the preferred substrate. In this case, Asf1 phosphorylation should increase when the level of soluble histones is low. We therefore investigated Asf1a phosphorylation status in cells experiencing a deficiency of new soluble histones. Since histones produced in S phase are rapidly incorporated into chromatin, short-term inhibition of protein synthesis by CHX is routinely used to reduce the pool of new soluble histones [41] , [42] . Asf1a phosphorylation, detected by the pS166 antibody or mobility shift, increased in S phase cells after short-term CHX treatment ( Fig. 6b ). Moreover, depletion of two key factors required for canonical histone biosynthesis, FLASH and SLBP [43] , [44] , also enhanced Asf1a phosphorylation in S phase ( Fig. 6b , Supplementary Fig. 7b ), substantiating the link between lack of soluble histones and TLK phosphorylation of Asf1. Asf1 is mainly found in the nucleus where it distributes into highly mobile (soluble) and chromatin-bound complexes [6] , [11] , [19] . We noted that hyper-phosphorylated Asf1a was enriched relative to the unphosphorylated form in chromatin when compared with the soluble fraction ( Fig. 6c ). Analysis of TLK1 revealed that a fraction of the kinase also remains in chromatin after extraction with Triton ( Fig. 6c ). Intriguingly, the level of chromatin-bound TLK1 increased when histone biosynthesis was impaired by short-term CHX treatment or FLASH/SLBP depletion ( Fig. 6d,e ). In contrast, TLK1 was released from chromatin in response to replication stress ( Fig. 6d ). Thus, TLK1 binding to chromatin correlates with Asf1 phosphorylation status ( Fig. 6b,d and e ). Asf1a pS166 could be detected in chromatin by western blot ( Fig. 6d ) but not by immunofluorescence. However, taking advantage of a GFP-TLK1 conditional cell line, we could address the localization of the kinase. As expected [34] , GFP-TLK1 was mainly nuclear. Yet, pre-extraction revealed two populations of cells; one with a diffuse nuclear signal and another showing distinct nuclear foci ( Supplementary Fig. 7c ). Co-staining with PCNA to mark replication sites revealed that non-S phase cells generally showed diffuse distribution of GFP-TLK1 in chromatin. In contrast, GFP-TLK1 localized in foci overlapping with PCNA replication patterns in the majority of S phase cells ( Fig. 6f ). Here we identify multiple TLK phosphorylation sites in human Asf1a and Asf1b ( Fig. 7a ) and provide evidence that phosphorylation stimulates the association of Asf1a with histones and downstream chaperones in vivo . We propose that TLK signalling promotes histone provision in S phase by targeting histone-free Asf1 and stimulating its ability to shuttle histones to sites of chromatin assembly ( Fig. 7b ). The key pieces of evidence in support of this model are (i) Asf1a phosphorylation is required for timely progression through S phase, (ii) phospho-mimetic Asf1a shows superior ability to form cellular complexes with histones and downstream chaperones, (iii) TLK1 binds to Asf1a via the same pocket as histone H3-H4 and (iv) TLK1 recruitment to chromatin and Asf1a phosphorylation is induced in cells experiencing deficiency of new histones. 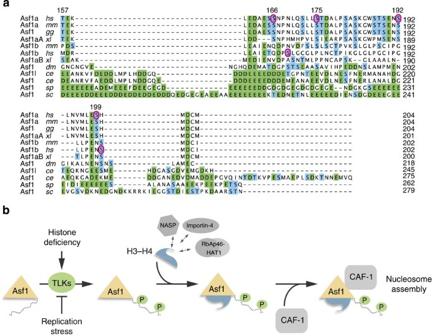Figure 7: Phosphorylation site conservation and model. (a) Sequence alignment of the Asf1 C-terminal tails performed by the ClustalW2 algorithm.Homo sapiens,hs;Mus musculus,mm;Gallus gallus,gg;Xenopus laevis,xl;Drosophila melanogaster,dm;Caenorhabditis elegans,ce;Saccharomyces cerevisiae,sc;Schizosaccharomyces pombe,sp. Acidic residues are indicated in green and Ser/Thr residues are in blue. Purple circles denote TLK1 phosphorylation sites in human Asf1a and Asf1b identified in this study. (b) Hypothetical model for how TLK phosphorylation fine-tunes Asf1-dependent histone provision during genome duplication. TLKs bind histone-free Asf1 and phosphorylate the tail at multiple sites. This in turn facilitates complex formation with histones and the downstream chaperones HIRA and CAF-1. TLK signalling responds to histone demand; Asf1a phosphorylation increases when cells lack new soluble histones and decreases if DNA synthesis is blocked and histones demand drops. Figure 7: Phosphorylation site conservation and model. ( a ) Sequence alignment of the Asf1 C-terminal tails performed by the ClustalW2 algorithm. Homo sapiens , hs ; Mus musculus , mm ; Gallus gallus , gg ; Xenopus laevis , xl ; Drosophila melanogaster , dm ; Caenorhabditis elegans , ce ; Saccharomyces cerevisiae , sc ; Schizosaccharomyces pombe , sp . Acidic residues are indicated in green and Ser/Thr residues are in blue. Purple circles denote TLK1 phosphorylation sites in human Asf1a and Asf1b identified in this study. ( b ) Hypothetical model for how TLK phosphorylation fine-tunes Asf1-dependent histone provision during genome duplication. TLKs bind histone-free Asf1 and phosphorylate the tail at multiple sites. This in turn facilitates complex formation with histones and the downstream chaperones HIRA and CAF-1. TLK signalling responds to histone demand; Asf1a phosphorylation increases when cells lack new soluble histones and decreases if DNA synthesis is blocked and histones demand drops. Full size image Most of the TLK1 phosphorylation sites we identify in human Asf1a and Asf1b are conserved in vertebrates ( Fig. 7a ). A few of these sites have been found in large phospho-proteomic analyses (S192, S166) [45] , [46] , and Asf1a S192 and Asf1b S198 were recently reported to be phosphorylated in vitro by TLK2 (ref. 40 ). It was proposed that S192 phosphorylation stabilizes Asf1a (but not Asf1b) by preventing proteasomal degradation [40] . We did not see changes in protein stability upon mutation of multiple Asf1a phosphorylation sites into either aspartic acids or alanines. However, we noticed that cycloheximide treatment stimulates phosphorylation of wild-type Asf1a considerably, which given the mobility shift of the phospho-forms may influence stability measurements. We also note that, while phosphorylation peaks in S phase, Asf1a protein levels remain relatively constant during the cell cycle [22] , [32] . Our data propose that TLK phosphorylation augments the ability of Asf1 to take up histones and engage with downstream chaperones when histone demand is high during replication. Since the acidic tail of S. cerevisiae Asf1 ( sc Asf1) contributes to histone binding and association with the heterotrimeric CAF-1 complex in vitro [26] , [29] , [31] , our results support the idea that TLK phosphorylation compensate for the lack of C-terminal acidic stretches in metazoan Asf1 homologues [33] . In yeast the tail confers an advantage to sc Asf1 in silencing [47] , but tailless sc Asf1 rescues the cell cycle defects and sensitivity to genotoxic stress of asf1 mutants [26] . Similarly, our data imply that TLK phosphorylation is not critical for Asf1 function, but makes it a more powerful histone chaperone better able to meet the demand for histones in S phase. Phosphorylation of the four C-terminal sites in Asf1a only moderately affects the charge of the full-length protein ( Supplementary Fig. 5d ), while the acidic tail of yeast Asf1 influences the pI substantially. However, considering the Asf1a tail alone, phosphorylation reduces the charge substantially and even more so than the phospho-mimetic mutations ( Supplementary Fig. 5d ). Our biochemical data show that multiple tail phosphorylations in Asf1a promote complex formation with histone H3-H4, histone-dependent partners like NASP and Importin-4, and the downstream chaperones HIRA and CAF-1. Similar to phospho-mimetic mutations, removal of the unmodified Asf1a tail augments histone binding in cells and cell extracts. Thus, the simplest model is that phosphorylation alleviates a negative effect of the unstructured tail. In addition, it is plausible that the phosphorylated tail might aid histone binding directly. We could not measure significant differences in binding rate constants for the interaction between histone H3-H4 and Asf1a wild-type, phospho-mimetic and tailless proteins. Nevertheless, wild-type Asf1 shows very high affinity towards H3-H4, which makes it challenging to identify a potential additional contribution of the acidic tail. Moreover, we cannot exclude that electrostatic immobilization of H3-H4 obstructs an interaction with the acid tail of phospo-mimetic Asf1. Further biophysical and structural studies are thus required to resolve exactly how phosphorylation enables Asf1 to bind histones more efficiently in a cellular context. Asf1a and Asf1b are found in complex with both histones H3.1-H4 and H3.3-H4 (ref. 20 ). Both histone variants can be deposited in S phase; the predominant replication-coupled pathway involves CAF-1 (refs 48 , 49 ), while HIRA contributes with gap-filling and histone replacement independent of replication [48] , [50] . Asf1a and Asf1b can both interact with CAF-1 (refs 15 , 20 ) and provide histones for replication-coupled nucleosome assembly [6] . In contrast, in vitro and in vivo data suggest that Asf1a would be the main histone donor for HIRA [20] , [21] , [23] . Phosphorylation does not appear to guide the choice of specific assembly pathway, as it enhances association of Asf1a with CAF-1 and HIRA as well as Asf1b binding to CAF-1. It remains unclear how histones are transferred to HIRA and CAF-1. Histone binding may itself promote Asf1 interaction with its downstream chaperones, as histone H3-H4 binding to sc Asf1 changes the B-domain binding pocket to facilitate interaction with CAF-1 p60 (Cac2) in vitro [29] . This would be consistent with the enhanced association of phospho-mimetic Asf1a with CAF-1 and HIRA in human cells, and explain why neither in vitro phosphorylated Asf1a nor the phospho-mimetic mutant show enhanced binding to recombinant CAF-1 p60 in vitro (ref. 15 , our unpublished results). Our SILAC analysis shows that phosphorylation does not increase the binding of Asf1a to Codanin-1, which also binds Asf1 via a B-domain and negatively regulates Asf1-H3-H4 nuclear import [51] . This suggests that phosphorylation is not beneficial for all B-domain containing binding partners but favours those that promote histone deposition. In vitro , sc CAF-1 and sc Asf1 do not reside together in a stable complex when both chaperones are bound to histones [29] . Consistent with this, Asf1 binding to CAF-1 in human cells is weak and lost upon high-salt washes (Jasencakova and Groth, unpublished). The simplest explanation for our observation is that phosphorylation favours formation of a complex where histone H3-H4 has not yet been transferred from Asf1 to CAF-1. The work of Liu and colleagues [29] suggests that Asf1 would be released once histone transfer takes place. Future studies should address the possibility that de-phosphorylation might trigger this event. Indeed, if phosphorylation promotes histone uptake and formation of a (H3-H4)-Asf1-CAF-1 complex, de-phosphorylation might in turn favour release of histones from Asf1. The assembly of newly synthesized DNA into nucleosomes is central for maintaining chromatin organization and genome integrity in dividing cells. The tight coupling of histone biosynthesis to DNA replication is well established [4] . Our data argue that TLK signalling provides an additional means to regulate histone provision. We find that TLK1 binding to Asf1 requires an intact histone-binding pocket, and, consistent with a mutually exclusive interaction, TLK1 can compete with histones for Asf1 binding in vitro [52] . Phosphorylation of Asf1 and/or TLK itself has been suggested to trigger their dissociation in vitro [37] . However, in cells the interaction appears to be dynamic and only kinase inactive TLKs form a stable complex with Asf1 (ref. 32 ). Recently, the S. cerevisiae checkpoint kinase Rad53 was shown to contact the histone-binding pocket in sc Asf1 (ref. 53 ). This analogy between TLKs and Rad53 is intriguing and supports the idea that, although TLKs do not share homology with Rad53, these kinases may have evolved as an extra regulatory layer replacing direct control of Asf1 function by checkpoint kinases. TLK activity is high in S phase when histone demand peaks, and is rapidly reduced by checkpoint signalling if replication is inhibited [35] and histone demand drops [6] . TLK activity would thus respond to ongoing DNA synthesis and histone demand in two ways; (i) via checkpoint signalling and (ii) by preferentially targeting histone-free Asf1. Consistent with this, Asf1a pS166 phosphorylation is enhanced in cells lacking new soluble histones for chromatin assembly and reduced in response to replication stress. Control of Asf1 phosphorylation by both checkpoints and histone pools probably explains why Chk1 inhibition alone is not sufficient to rescue Asf1 phosphorylation in HU treated cells. TLK binding to chromatin correlates with Asf1a pS166 in response to stresses such as depletion of nucleotide and soluble histone pools. Moreover, TLK1 is present at sites of ongoing replication. We thus speculate that Asf1 phosphorylation could, at least in part, take place in chromatin at replication sites. The simplest scenario would be that Asf1, once it has delivered its histone cargo to CAF-1, becomes a target for TLK phosphorylation, which in turn fuels recruitment of additional histones to active replication forks. Lack of TLK function leads to severe chromatin defects in flies and worms [37] , [38] , and TLK mutations jeopardize gene silencing in plants [54] . Our work proposes that TLK signalling ensures efficient histone delivery during genome duplication, hereby facilitating proper restoration of the epigenetic landscape. An exciting perspective for future research is that TLKs might target additional factors involved in chromatin replication and coordinate a cellular response to histone demand. Cloning Plasmids used in this study are listed in Supplementary Table 1 . Human Asf1 was inserted in frame into pcDNA5/FRT/TO-FLAG-HA [51] . QuickChange Site-Directed Mutagenesis (Stratagene) was used to generate Asf1a mutants 4D (S166D, S175D, S192D, S199D), 4A (S166A, S175A, S192A, S199A), 3A (S166A, S175A, S192A), 2A (S166A, S175A), and Asf1b mutants 2E (S169E, S198E), Asf1b 2A (S169A, S198A), 1A (S198A). All constructs were verified by sequencing. Cell culture and transfections Cell lines are listed in Supplementary Table 2 . U-2-OS and Hela S3 cell lines were grown in DMEM (Gibco) supplemented with penicillin/streptomycin, 10% FBS (Hyclone) and drugs for selection (see Supplementary Table 2 ). HeLa S3 cells stably expressing OneStrep-tagged Asf1 (a and b) were described [19] , [51] . Asf1-inducible cell lines were generated in U-2-OS Flp-In T-Rex (Invitrogen) as single-cell clones. TLK1-inducible cell lines were generated as described [35] . For expression of FLAG-HA-Asf1a (e-Asf1a) wild-type (wt) and mutants, cells were induced with 1 μg ml −1 tetracycline for 8 to 14 h. For expression of GFP-TLK1, cells were induced for 24 h. Expression plasmids were introduced by FuGENE 6 (Promega) transfection or by electroporation using a GenePulser Xcell (BIO-RAD). Cells were transfected with siRNAs at 100 nM concentration using Oligofectamine (Invitrogen). The Asf1 (a and b) targeting siRNAs were described [19] , siRNAs against FLASH (sense strand 5′-CCGCAAGGAUGAAGAAAUAdTdT-3′) and SLBP (sense strand 5′-GGAUGUGAUUUGCAAGAAAdTdT-3′) were from Sigma. DNA content was analysed by propidium iodide staining on a FACScalibur (BD) using CellQuest Pro 6.0 software (BD). Cell cycle profiles were generated by FlowJo 8.8.4 software (Tree Star) and quantified by Dean-Jett-Fox model and manual gating. Cells were synchronized by a single thymidine (Sigma, 2 mM) block for 17 h ( Fig. 3e ) or hydroxyurea (Sigma, 3 mM) for 20 h ( Fig. 3d ) and released into fresh media with deoxycytidine (Sigma, 24 μM). Where indicated, cells were treated with HU (3 mM, 1 h), UCN-01 (300 nM, 1 h) or CHX (50 μg ml −1 , from 1 to 4 h; all from Sigma). UCN-01 was added 15 min before HU. Complex purification and gel-filtration Purification of OneStrep-Asf1a/b complexes for mass spectrometry analysis from cytosolic and nuclear extracts was performed essentially as described [11] , [51] using high-stringency washes (see below). Cytosolic and nuclear extracts for isolation of the e-Asf1a complexes were prepared as described [11] . In brief, cells were washed with ice-cold PBS, swollen in buffer E (20mM Hepes-KOH pH 7.8, 5mM potassium acetate, 0.5mM MgCl 2 ) supplemented with inhibitors (1 mM DTT, 10 μg ml −1 leupeptin, 10 μg ml −1 pepstatin, 0.1 mM PMSF, 0.2 mM sodium vanadate, 5 mM sodium fluoride, 10 mM beta-glycerolphosphate). Cells were homogenized using loose type pestle. Pelleted nuclei (1,500 g, 5 min) were extracted with 2.5 × volume of extraction buffer N (buffer E with inhibitors, 540 mM NaCl, 10% glycerol). Extracts were pre-cleared with agarose beads (SuperFlow 6, IBA) for 1 h, followed by 2 h incubation with anti-FLAG M2-agarose beads (Sigma). We used low-stringency washes for isolation of nuclear complexes (Buffer A: 150 mM NaCl, 50 mM Tris pH 7.8, 0.2 mM EDTA, 0.2% NP-40, 1 mM DTT, 5% glycerol, protease and phosphatase inhibitors) and high-stringency washes (buffer A, containing 500 mM NaCl) for purification of cytosolic complexes. Complexes were eluted from the beads with a FLAG-peptide (400 μg ml −1 ). FLAG-HA-Asf1b complexes were isolated under low stringency using anti-FLAG beads from whole-cell extracts (300 mM NaCl, 0.5% NP-40, 50 mM Tris pH 7.5, 0.2 mM EDTA, 5% glycerol and inhibitors). For fractionation of cells by triton extraction ( Fig. 6c–e ), soluble proteins were extracted in CSK-T (10 mM PIPES pH 7, 100 mM NaCl, 300 mM sucrose, 3 mM MgCl2, 0.5% Triton, inhibitors) for 8 min before the pellet was isolated and washed once in CSK-T. Total cell lysates ( Figs 1f , 2a , 3a ) were made in Laemmli sample buffer (LSB: 50 mM Tris pH 6.8, 100 mM DTT, 2% SDS, 7.5% glycerol, bromphenol blue) and treated with Benzonase (Novagen) for 30 min at room temperature. Gel filtration analysis of mid-S phase cytosolic extract from inducible U-2-OS cells expressing similar levels e-Asf1a wt/4D/4A was performed as described [6] , [51] with minor modifications. In brief, 1 mg of extracts was loaded on SuperdexG200 10/300 GL column (GE Healthcare) and complexes were eluted in buffer E containing 100 mM NaCl, 5% glycerol and inhibitors at a flow of 0.3 ml min −1 in 400 μl fractions. Proteins were precipitated by trichloroacetic acid and Na deoxycholate and analysed by western blotting with Gel Filtration Calibration Kit HMW (high molecular weight, GE Healthcare) as a size marker. Antibodies Asf1a pS166 rabbit polyclonal antibodies were generated against Asf1a phospho-peptide (CTEKLEDAESpSNPNL) and double affinity purified (Genscript). TLK1 (‘TALAF’) rabbit polyclonal antibodies were generated against the peptide KKKSPTALAFGDHPIVQPKQLSFK. Primary antibodies and dilutions are listed in Supplementary Table 3 . Secondary antibodies (anti-mouse (115-035-068, 1:20,000), anti-rabbit (711-035-152, 1:20,000) and anti-rat (122-035-068, 1:20,000)) conjugated with HRP were from Jackson ImmunoResearch Labs; anti-rabbit-Alexa488 (1:1,000) and anti-mouse-Alexa568 (1:1,000) were from Invitrogen. Full scans of all western blots are included in Supplementary Figs 8–10 . For quantification of western blots, films were scanned and signal intensities were analysed with NIH Image J 1.41. In vitro kinase reactions Recombinant myc-TLK1 wild-type (wt) or kinase-inactive (ki) were purified from Sf9 insect cells infected with recombinant baculovirus [34] , using protein G sepharose beads (GE Healthcare) coupled to myc antibodies. Myc-TLK1 was eluted in low pH buffer (100 mM glycin pH 2.5, 1 mM DTT, 2.5 mM NaF), and pH was adjusted by addition of 1M Tris pH 8.0 (supplemented with 1 mM DTT, 2.5 mM NaF). In vitro TLK1 kinase assays were performed essentially as described [34] , [35] . In brief, myc-TLK1 was incubated in 25 μl kinase assay buffer (KAB - 50 mM HEPES pH 7.2, 10 mM MgCl 2 , 5 mM MnCl 2 , 2.5 mM EGTA, 1 mM DTT, 1 mM NaF, 10 μM ATP, 10μCi/μl [γ32P]-ATP) with 1 μg GST-Asf1a for 30 min and 30 °C. Kinase reactions were stopped by the addition of 4xLSB, and reaction products were resolved on a 12% SDS-PAGE. [ 32 P] incorporation was quantified on a PhosphorImager FLA3000 (Fujifilm, Tokyo). For identification of TLK1 phospho-sites in Asf1 (a and b) by mass spectrometry, the kinase reaction contained 50 μM ATP, 6μg of recombinant Asf1 (a or b) and myc-TLK1 (2 μg). Reaction products were resolved on a 15% SDS-PAGE gel and stained with Coomassie Blue. Slow-migrating bands were cut and analysed by LC-MS/MS. Protein purification and pull-down assays GST-Asf1 fusion proteins were expressed in E. coli and purified on glutathione-Sepharose beads 4B (GE Healthcare Life Science) using buffer containing 20 mM Tris–HCl pH 8, 500 mM NaCl, 0.1% Triton X100, 0.5 mg ml −1 Lysosyme and protease inhibitors [32] . Proteins were eluted from the glutathione-Sepharose beads with 20 mM Gluthathion (GE Healthcare Life Science) in elution buffer (100 mM Tris–HCl pH 8, 120 mM NaCl, 0.1% Triton X100, 10% Glycerol and proteinase inhibitors). Where indicated, Asf1 was cleaved from GST with PreScission protease (GE Healthcare). For in vitro binding, myc-TLK1 wt or ki on anti-myc sepharose beads were incubated with Asf1a proteins for 2 h at 4 °C in buffer A. The reactions were washed five times with buffer A, and bound proteins were solubilized in Laemmli sample buffer (4xLSB: 200 mM Tris pH 6.8, 400 mM DTT, 8% SDS, 30% glycerol, bromphenol blue). For GST pull-downs, GST-Asf1a proteins were coupled to glutathione-sepharose beads (GE Healthcare) for 1 h at 4 °C and incubated with cell extracts in buffer A for 3 h at 4 °C. Reactions were washed six times with buffer A and bound proteins were solubilized in LSB. Where indicated, GST-Asf1a was phosphorylated by myc-TLK1 wt or ki before pull-down reactions. After the kinase reaction, GST proteins were separated from myc-TLK1-beads by centrifugation. Mass spectrometric analyses of Asf1 phosphorylation sites Asf1a and Asf1b gel bands were subjected to in-gel digestion as previously described [55] , with replicate bands digested with either 100 ng of trypsin (overnight at 37 °C) or thermolysin (Calbiochem, 60 min at 56 °C). Phosphopeptide enrichment was performed on titanium dioxide microcolumns before the resulting eluates were desalted with Poros R3 material [56] , [57] . LC-MS/MS was conducted on an EASY-nLC system (Thermo Fisher Scientific) coupled to an LTQ-Orbitrap XL mass spectrometer (Thermo Fisher Scientific) as reported [58] , with a minimum threshold of 30,000 precursor ions required to trigger MS/MS spectrum acquisition. Using Proteome Discoverer 1.0 software (Thermo Fisher Scientific), raw data files were submitted to Mascot database searches 2.2.04 (Matrix Science). An NCBI non-redundant database (20090412) containing 222,460 human protein sequences was searched with the following parameters: ESI-TRAP was selected as the instrument type, with specified mass tolerances of 10 p.p.m. (precursor) and 0.6 Da (fragment). N-terminal protein acetylation, methionine oxidation and phosphorylation (serine, threonine and tyrosine) were set as variable modifications. Cysteine carbamidomethylation was included as a fixed modification. Thermolytic searches were permitted up to nine missed cleavages, with cleavage specificity set N-terminal to valine, isoleucine, leucine, phenylalanine, alanine and methionine. Tryptic searches were conducted with one missed cleavage permissible. Only Asf1a and Asf1b phosphopeptides with Mascot ion scores above 20 were considered for evaluation, which involved manual validation of the MS/MS spectrum to determine the site of phosphorylation. The Asf1 phosphopeptide mass spectrometry data have been deposited to the ProteomeXchange Consortium ( http://www.proteomexchange.org ) via the PRIDE partner repository [59] with the data set identifier PXD000686. SILAC-based proteomics For SILAC ( S table I sotope L abelling with A mino acids in C ell culture), conditional cell lines expressing e-Asf1a wt and phospho-mimetic (4D) mutants were grown in medium depleted for Arginine and Lysine (Thermo Scientific, RPMI 1640) and supplemented with dialysed FBS (Invitrogen, 26400-036), MEM non-essential amino acids (Invitrogen, 11140) and Glutamax (Invitrogen, 35050-038). SILAC medium for e-Asf1a wt cells was complemented with 66 mg l −1 of arginine and 100 mg l −1 of lysine (light, Arg0/Lys0, Sigma), while medium for e-Asf1 4D cell lines was complemented with heavy lysine and arginine (Arg6/Lys8, Cambridge lab, CNLM-291-0.25, CLM-2265-0). Cells were maintained for 8 to 9 divisions in heavy or light medium before analysis. e-Asf1a wt and 4D were expressed at a similar level and complexes were isolated under low-stringency conditions (buffer A) from whole-cell extracts. Before elution from the FLAG M2 beads, e-Asf1a wt and 4D complexes were mixed 1:1. Eluted proteins were run on SDS-PAGE, excised from the gel and subjected to LC-MS/MS. In-gel digestion was performed as described [55] , except chloroacetamide was used in place of iodoacetamide as the alkylating agent [60] . LC-MS/MS was executed with an EASY-nLC system coupled to an Q Exactive mass spectrometer (Thermo Fisher Scientific) using the 76 min ‘sensitive’ method as previously described [61] with a 2 Da isolation width. Data files (technical duplicates) were processed with MaxQuant 1.2.7.1, with searches conducted against a UniProt database containing 86875 human protein sequences (2012_06) concatenated with reverse entries and a list of protein sequences from commonly observed contaminants. The enzyme specificity was set to trypsin/P with a maximum of two miscleavages allowed. Recalibrated spectra were searched with a 6 p.p.m. MS tolerance and 20 p.p.m. MS/MS tolerance. A false discovery rate of 1% was employed for protein and peptide identifications, with a minimum of two peptides required for each protein identification. Criteria for peptide identification included a minimum score of 60 and a minimum peptide length of six amino acids. For protein quantification, a minimum of two ratio counts was required. Immunostaining Cells were either pre-extracted with 0.5% Triton in CSK buffer (10 mM PIPES pH 7, 100 mM NaCl, 300 mM sucrose, 3 mM MgCl2) for 5 min at 4 °C to remove soluble proteins or fixed directly with 4% formaldehyde (10 min at room temperature) and permeabilized with 0.2% Triton. To reveal the epitope recognized by the PCNA antibody, cells were treated with methanol for 20 min at −20 °C. EdU labelling (40 μM, 20 min) was detected by Click-iT Cell Reaction (Invitrogen). Fluorescence images were collected on a DeltaVision system and analysed by SoftWoRX 5.0.0 or on a Zeiss inverted microscope Axiovert 200 M equipped with LSM510 Laser module with a 63x objective (C-APOCHROMAT, water immersion, 63−/1.2W Korr). Brightness and contrast were adjusted using Adobe Photoshop CS5 (12.0.4). Surface plasmon resonance Human recombinant H3.1-H4 tetramers (NEB, M2509S) were diluted 200-fold to 50 nM in running buffer (10 mM Tris pH 7.8, 100 mM NaCl, 50 μM EDTA, 0.5 mM DTT and 0.05% (v/v) P-20) to promote the dissociation into H3.1-H4 heterodimers [62] . H3.1-H4 was non-covalently captured by electrostatic interaction directly onto one of the flow cells in a C1 Sensor Chip (GE Healthcare) by a 225 s injection at 10 μl min −1 followed by a 17 min washing step with running buffer at 20 μl min −1 to attenuate further decay of the captured surface during the subsequent kinetic experiment. Monomeric status of recombinant Asf1a (cleaved from GST-tag) was confirmed by size exclusion chromatography (SuperdexG200 5/150 GL). Next, Asf1a preparations (1–73 nM dilutions in running buffer) were allowed to interact with the H3.1-H4 captured on the surface and with matched un-captured control surface for 200 s before the dissociation phase was recorded for 45 min. The surface was regenerated by two consecutive 30 s injections of 0.3% (w/v) SDS. All measurements were performed with a flow rate of 20 μl min −1 at 20 °C using a BiaCoreT200 (GE Healthcare). The recorded data were processed by double referencing using the paired buffer runs analysed immediately before the sample injection. Kinetic rate constants for the interactions were derived by local fitting double referenced data to a simple bimolecular interaction model using the BiaEvaluation 4.1 software. Statistical analysis Data were subjected to a two-tailed Student’s t -test to resolve statistical significance (Prism 5.0). Results from at least three independent experiments are presented and error bars indicate s.d. Accession codes : The Asf1 phosphopeptide mass spectrometry data is available from the ProteomeXchange Consortium under the data set identifier PXD000686. How to cite this article: Klimovskaya, I. M. et al. Tousled-like kinases phosphorylate Asf1 to promote histone supply during DNA replication. Nat. Commun. 5:3394 doi: 10.1038/ncomms4394 (2014).